The NF-YC–RGL2 module integrates GA and ABA signalling to regulate seed germination inArabidopsis The antagonistic crosstalk between gibberellic acid (GA) and abscisic acid (ABA) plays a pivotal role in the modulation of seed germination. However, the molecular mechanism of such phytohormone interaction remains largely elusive. Here we show that three Arabidopsis NUCLEAR FACTOR-Y C (NF-YC) homologues NF-YC3, NF-YC4 and NF-YC9 redundantly modulate GA- and ABA-mediated seed germination. These NF-YCs interact with the DELLA protein RGL2, a key repressor of GA signalling. The NF-YC–RGL2 module targets ABI5 , a gene encoding a core component of ABA signalling, via specific CCAAT elements and collectively regulates a set of GA- and ABA-responsive genes, thus controlling germination. These results suggest that the NF-YC–RGL2–ABI5 module integrates GA and ABA signalling pathways during seed germination. Seed germination is an essential developmental process in the life cycle of higher plants. Plants start with the release of seeds dormancy and launch of germination when the circumstance is favourable for growth, and subsequently, the seedling is established and developing, which serves as the basis for species propagation and agricultural production [1] , [2] . Germination includes a series of sophisticated biochemical reactions tightly regulated by environmental and intrinsic cues such as light irradiation, temperature, water uptake and change of endogenous phytohormone levels, which compose the necessary events to trigger specific signalling for the transition from embryonic to vegetative development [1] , [3] . Germination process is principally controlled by the phytohormone balance of gibberellic acid (GA) and abscisic acid (ABA), which have antagonistic effects on this vital developmental phase [4] , [5] . GA is one of most important phytohormones that coordinates with a cascade of molecular signalling regulation to promote seed germination [6] . The essential role of GA on germination initiation is best illustrated by previous reports that GA-deficient mutant ga1 fails to germinate without exogenous GA [7] , [8] . Conversely, ABA counteracts the effect of GA during seed germination by inhibiting water uptake and endosperm rupture rather than testa rupture [9] , [10] . Identification of the ABA-related mutants in Arabidopsis has also provided important evidences to reveal the effect of ABA on GA-mediated seed germination. For example, the ABA synthesis-defective mutants aba1 and aba2 are able to rescue the non-germinating phenotype of ga1 (refs 11 , 12 , 13 ), supporting the antagonistic roles of ABA and GA during seed germination process. DELLA proteins serve as the key repressors in GA signalling pathway to modulate plant growth and development. In Arabidopsis , five DELLA family members, GA-INSENSITIVE (GAI), REPRESSOR OF ga1-3 (RGA), RGA-LIKE 1 (RGL1), RGL2 and RGL3, share the conserved DELLA motif and display redundant and distinct roles under the control of GA receptor-mediated degradation [14] , [15] , [16] , [17] , [18] . Among them, RGL2 has been considered as the major negative regulator in the light-dependent seed germination since loss of function of RGL2 is sufficient to suppress the non-germinating phenotype of the ga1 mutant [16] , [19] , [20] . In addition, several studies revealed that a bZIP transcriptional factor ABA INSENSITIVE 5 (ABI5), the central ABA signalling component which directly regulates the late embryonic and abundant (LEA) genes including EM1 and EM6 , might serve as the final downstream repressor of seed germination in the counterbalance of ABA and GA signals [21] , [22] , [23] . When GA levels are low, the accumulation of RGL2 leads to an increase in endogenous ABA levels by activating the expression of XERICO gene that encodes an unknown RING-H2 zinc finger protein involved in ABA synthesis, in turn elevates ABI5 transcription and protein levels, thus inhibiting seed germination [23] , [24] , [25] . Although studies have suggested a significant crosstalk of GA and ABA signalling during seed germination, the detailed mechanism of antagonism between these two phytohormones by which the plants precisely modulate germination remains elusive. The NUCLEAR FACTORY C proteins (NF-YCs), are structurally characterized by a histone-fold domain (HFD) and closely related to the core histone H2A, functionally act as one subunit of the NF-Y heterotrimer transcriptional factor that specifically recognizes the CCAAT-box in eukaryotes [26] , [27] . In plants, NF-YCs function as important participants in various developmental and stress responses including flowering control [28] , [29] , [30] and abiotic stress resistance [31] , [32] , [33] , [34] . Recently, studies demonstrated that NF-YCs are also involved in the regulation of phytohormone response [35] , [36] . The diverse roles of NF-YCs, together with those of another two NF-Y subunits NF-YA and NF-YB, imply the widely flexible formation of NF-Y complex that are spatially and temporally regulated by various developmental and growth conditions [27] , [37] . In this study, we showed that three NF-YC homologues NF-YC3, NF-YC4 and NF-YC9 are engaged redundantly in the suppression of GA-mediated seed germination through directly interacting with the DELLA protein RGL2, a major GA signalling repressor in germination. Further genome-wide transcriptome analysis reveals that the NF-YC–RGL2 module integrates GA and ABA signalling to converge at a set of GA- and ABA-responsive genes. Notably, NF-YCs and RGL2 were showed to directly regulate ABI5 gene expression regardless of ABA synthesis via recognizing two specific CCAAT elements in the ABI5 promoter. Consistently, the ABA-mediated germination inhibition is attenuated in the null mutants of NF-YCs and RGL2 , suggesting that NF-YC and RGL2 are required for ABA-mediated seed germination. These findings establish that NF-YCs, together with DELLAs, act as the critical joint modulators to synergistically mediate the antagonism of GA and ABA, providing a new insight into understanding towards phytohormones fine-tuning in seed germination in plants. NF-YC homologues repress GA-mediated seed germination We previously revealed that NF-Y complex regulates flowering time under GA pathway [36] . As GA-mediated molecular response is critical for seed germination, to investigate the role of Arabidopsis NF-Y genes in germination, we compared the germination rates of the diverse NF-Y mutant seeds in either the presence or absence of the GA biosynthesis inhibitor paclobutrazol (PAC), respectively. Intriguingly, nf-yc3 nf-yc4 nf-yc9 ( nf-ycT ), the combinatorial null mutant of the closest homologues NF-YC3 , NF-YC4 and NF-YC9 in Arabidopsis NF-YC subfamily, similar to the key GA-related germination repressor mutant rgl2 (ref. 16 ), showed a strong resistance to PAC, but it has no difference in germination rate with the wild-type under mock treatment ( Fig. 1a,b ). By contrast, there was no significant difference in germination performance between the single or double mutants of NF-YC3 / 4 / 9 and the wild type ( Supplementary Fig. 1a,b ). These results suggest redundant roles of NF-YC3 , NF-YC4 and NF-YC9 in repression of the GA-mediated seed germination. Consistently, the seeds of 35S:NF-YC3 and 35S:NF-YC9 exhibited lower germination rates than the wild type in the presence of a low concentration (0.5 μM) of PAC ( Supplementary Fig. 1c,d ). The analysis of gradient PAC concentrations further confirmed that 35S:NF-YC9 was hypersensitive, and nf-ycT showed reduced sensitivity to PAC, in comparison with the wild type ( Fig. 1c ). Given that stratification increases Arabidopsis seeds sensitivity to GA during germination [38] , we also examined germination phenotype of nf-ycT mutant in the absence of stratification. Similar to those with stratification, nf-ycT seeds showed significant resistance to PAC as rgl2 under non-stratification conditions ( Supplementary Fig. 2 ). These results indicated that NF-YC homologues negatively regulate GA-mediated seed germination. 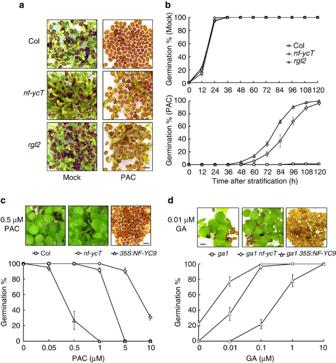Figure 1: NF-YCs inhibit GA response in seed germination. (a) Loss of function of threeNF-YChomologues orRGL2decreases the sensitivity of seeds germination to PAC. Germination phenotypes ofnf-yc3-2 nf-yc4-1 nf-yc9-1(nf-ycT),rgl2and the wild-type (Col) seeds were observed at 96 HAS (hour after stratification) on 1/2 MS medium containing 5 μM PAC or mock, respectively. (b) Statistic analysis of germination rate innf-ycT,rgl2and the wild-type seeds. The seeds were treated as described inaand the germination rates were recorded every 12 h until 120 HAS. (c) Overexpression ofNF-YC9seeds increases the sensitivity of seeds germination to PAC. Upper panel shows germination phenotypes of Col,nf-ycTand35S:NF-YC9#1seeds observed at 120 HAS on 1/2 MS medium containing 0.5 μM PAC. Lower panel shows germination rates of these seeds in response to different concentrations of PAC that were recorded at 120 HAS. (d) Loss of function of NF-YCs or overexpression ofNF-YC9affects the sensitivity of seeds inga1background to GA. Upper panel shows germination phenotypes ofga1,ga1 nf-ycTandga1 35S:NF-YC9seeds observed at 120 HAS on 1/2 MS medium containing 0.01 μM GA. Lower panel shows germination rate of these seeds in response to different concentrations of GA that were recorded at 120 HAS. All data represent mean±s.d. of at least 100 seeds. Scale bar, 1 mm. Figure 1: NF-YCs inhibit GA response in seed germination. ( a ) Loss of function of three NF-YC homologues or RGL2 decreases the sensitivity of seeds germination to PAC. Germination phenotypes of nf-yc3-2 nf-yc4-1 nf-yc9-1 ( nf-ycT ), rgl2 and the wild-type (Col) seeds were observed at 96 HAS (hour after stratification) on 1/2 MS medium containing 5 μM PAC or mock, respectively. ( b ) Statistic analysis of germination rate in nf-ycT , rgl2 and the wild-type seeds. The seeds were treated as described in a and the germination rates were recorded every 12 h until 120 HAS. ( c ) Overexpression of NF-YC9 seeds increases the sensitivity of seeds germination to PAC. Upper panel shows germination phenotypes of Col, nf-ycT and 35S:NF-YC9#1 seeds observed at 120 HAS on 1/2 MS medium containing 0.5 μM PAC. Lower panel shows germination rates of these seeds in response to different concentrations of PAC that were recorded at 120 HAS. ( d ) Loss of function of NF-YCs or overexpression of NF-YC9 affects the sensitivity of seeds in ga1 background to GA. Upper panel shows germination phenotypes of ga1 , ga1 nf-ycT and ga1 35S:NF-YC9 seeds observed at 120 HAS on 1/2 MS medium containing 0.01 μM GA. Lower panel shows germination rate of these seeds in response to different concentrations of GA that were recorded at 120 HAS. All data represent mean±s.d. of at least 100 seeds. Scale bar, 1 mm. Full size image Previous studies have shown that the GA-deficient mutant ga1 fails to germinate, which can be sufficiently recovered by exogenous GA or loss of function of RGL2 (refs 7 , 16 ). Considering that the similar observations on the nf-ycT and rgl2 mutants, and as a P450 enzyme inhibitor, PAC might have undesirable effect on other metabolic pathways including potentially increasing ABA levels through inhibition of ABA catabolism [39] , [40] , we thus examined whether NF-YCs could also affect ga1 germination as RGL2. Consistent with previous report [41] , different concentrations of GA gradually increased the germination rate of ga1 . nf-ycT significantly increased GA responsiveness in ga1 , whereas overexpression of NF-YC9 decreased that in ga1 ( Fig. 1d ). Further observations showed that, besides of nf-ycT , the NF-YC double mutants also partially rescued ga1 phenotype although the nf-yc single mutants had less effect on that ( Supplementary Fig. 3a,b ). Combined with that NF-YC3 , NF-YC4 and NF-YC9 genes expressed in germinating seeds ( Supplementary Fig. 4 ), these results support that Arabidopsis NF-YC3, NF-YC4 and NF-YC9 redundantly function as negative regulators in GA-mediated seed germination. NF-YCs interact with RGL2 The analogous genetic roles of NF-YCs and RGL2 prompted us to investigate whether NF-YCs functionally associate with RGL2 to regulate seed germination. We first found that AD-RGL2 interacted with BD-NF-YC3, BD-NF-YC4 and BD-NF-YC9 in yeast, respectively ( Fig. 2a ). Glutathione S-transferase (GST) pull-down assays showed that each His-NF-YC was precipitated by GST-RGL2 but not by GST alone ( Fig. 2b ), indicating the physical interaction between RGL2 and NF-YCs in vitro . Because NF-YC9-3FLAG fully rescued the PAC reduced-sensitivity phenotype of nf-yc9 and nf-ycT ( Supplementary Fig. 5 ), we thus focused NF-YC9 as representative of NF-YC homologues for further investigation. 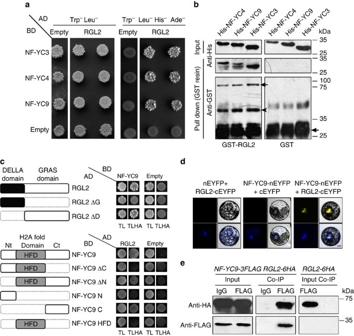Figure 2: NF-YCs interact with RGL2in vitroandin vivo. (a) Yeast two-hybrid assays show the interactions between RGL2 and NF-YCs. Transformed yeast cells were grown on SD/-Trp/-Leu/-His/-Ade and SD/-Trp/-Leu medium. (b) Pull-down assays show the direct interaction between His-NF-YCs and GST-RGL2 fusion proteinsin vitro. His-NF-YC proteins were incubated with immobilized GST or GST-RGL2 proteins, and immunoprecipitated fractions were detected by anti-His and anti-GST antibodies, respectively. Arrows indicate the specific bands of GST-RGL2 or GST, while arrowhead indicates the nonspecific bands. (c) Sketches show the domains of NF-YCs and RGL2 and their various deletions. Yeast two-hybrid assays show the interactions between RGL2, NF-YCs and their derivatives. Transformed yeast cells were grown on SD/-Trp/-Leu/-His/-Ade (TLHA) and SD/-Trp/-Leu (TL) medium. (d) BiFC analysis of interaction between NF-YC9-nEYFP and RGL2-cEYFP inArabidopsismesophyll protoplast. DAPI staining was used as the nucleus indicator. Scale bar, 10 μm. (e)In vivointeraction of NF-YC9 and RGL2 inArabidopsis. Plant nuclear extracts from PAC-treated seeds ofnf-yc9 NF-YC9:NF-YC9-3FLAG rgl2 pRGL2:RGL2-6HAwere immunoprecipitated by either anti-FLAG antibody or preimmune serum (IgG). The co-immunoprecipitated proteins were detected by anti-FLAG and anti-HA antibodies. Figure 2: NF-YCs interact with RGL2 in vitro and in vivo . ( a ) Yeast two-hybrid assays show the interactions between RGL2 and NF-YCs. Transformed yeast cells were grown on SD/-Trp/-Leu/-His/-Ade and SD/-Trp/-Leu medium. ( b ) Pull-down assays show the direct interaction between His-NF-YCs and GST-RGL2 fusion proteins in vitro . His-NF-YC proteins were incubated with immobilized GST or GST-RGL2 proteins, and immunoprecipitated fractions were detected by anti-His and anti-GST antibodies, respectively. Arrows indicate the specific bands of GST-RGL2 or GST, while arrowhead indicates the nonspecific bands. ( c ) Sketches show the domains of NF-YCs and RGL2 and their various deletions. Yeast two-hybrid assays show the interactions between RGL2, NF-YCs and their derivatives. Transformed yeast cells were grown on SD/-Trp/-Leu/-His/-Ade (TLHA) and SD/-Trp/-Leu (TL) medium. ( d ) BiFC analysis of interaction between NF-YC9-nEYFP and RGL2-cEYFP in Arabidopsis mesophyll protoplast. DAPI staining was used as the nucleus indicator. Scale bar, 10 μm. ( e ) In vivo interaction of NF-YC9 and RGL2 in Arabidopsis . Plant nuclear extracts from PAC-treated seeds of nf-yc9 NF-YC9:NF-YC9-3FLAG rgl2 pRGL2:RGL2-6HA were immunoprecipitated by either anti-FLAG antibody or preimmune serum (IgG). The co-immunoprecipitated proteins were detected by anti-FLAG and anti-HA antibodies. Full size image To identify whether the functional domains are required for the NF-YC and RGL2 interaction, the various truncated versions of RGL2 and NF-YC9 were used in yeast two-hybrid assays ( Fig. 2c ). The results showed that deletion of the GRAS domain [42] (RGL2ΔG) prevented RGL2 binding to NF-YC9, whereas deletion of the RGL2 amino-terminal (RGL2ΔD) which excluded the entire DELLA domain did not affect the interaction between RGL2 and NF-YC9 ( Fig. 2c ). On the other hand, RGL2 interacted with full length of NF-YC9 and deletion of the amino-terminal (NF-YC9ΔN) but not with the HFD [26] and the amino-terminal fragment (NF-YC9N) of NF-YC9 ( Fig. 2c ), indicating the carboxy-terminal fragment of NF-YC9 is necessary for interacting with RGL2 at least, although it alone revealed a self-activation in yeast. Therefore, these results suggest that the GRAS domain of RGL2 and carboxy-terminal of NF-YC9 contribute to interaction between RGL2 and NF-YC9, and may be indispensible components in potential biological function of this heterodimer. We next performed bimolecular fluorescence complementation (BiFC) analysis to examine the interaction between NF-YC9 and RGL2 in plants. The results showed that the interaction fluorescence of NF-YC9-nEYFP with RGL2-cEYFP existed in the cell nuclei, but no YFP signal was detected in the negative control ( Fig. 2d ). To perform co-immunoprecipitation assay, we further created nf-yc9 rgl2 pNF-YC9:NF-YC9-3FLAG pRGL2:RGL2-6HA homozygous lines in which NF-YC9-3FLAG expressed at comparable levels in the germinating seeds with mock and PAC treatment, whereas RGL2-6HA was only detected in those with PAC ( Supplementary Fig. 6 ). Both NF-YC9 and RGL2 fusion proteins retained the biological function in seeds as they are able to rescue the PAC reduced-sensitivity phenotype of mutants ( Supplementary Fig. 5 ). The co-immunoprecipitation results of PAC-treated nf-yc9 rgl2 pNF-YC9:NF-YC9-3FLAG pRGL2:RGL2-6HA seeds further confirmed the in vivo binding of NF-YC9 to RGL2 ( Fig. 2e ). Taken together, these data consistently support the direct interactions between the three NF-YC homologues and RGL2 proteins. Among DELLAs, RGL2 has been reported as the predominant repressor, and RGA, GAI and RGL1 play minor roles in GA-mediated seed germination in Arabidopsis L er ecotype [16] , [19] . Our observations confirmed that the non-germinating phenotype of ga1 was also partially suppressed by loss of RGA function or completely rescued by the rga rgl2 double mutant in Arabidopsis Col ecotype ( Supplementary Fig. 7a ). Consistent with this, like RGL2, RGA was shown to interact with NF-YC3, NF-YC4 and NF-YC9 in yeast, respectively ( Supplementary Fig. 7b ), which implies widespread interactions between NF-YCs and DELLAs. NF-YCs and RGL2 interdependently regulate seed germination The interaction between NF-YCs and RGL2 in plants suggests that these proteins may function together to regulate seed germination. To verify this hypothesis, we created various combinatorial genetic backgrounds of NF-YC and RGL2 by intercrossing. Investigations of germination rate showed that rgl2 fully suppressed the hypersensitivity of 35S:NF-YC9 to PAC ( Fig. 3a,b ). Consistently, although 35S:NF-YC9 enhanced the germination inhibition of ga1 at low GA condition (0.01–1 μM), it did not suppress ga1 germination at higher GA level (10 μM GA; Fig. 1d ). In addition, 35S:NF-YC9 also rarely affected germination of seeds grown in normal condition ( Fig. 3 ). Since RGL2 proteins are highly accumulated in ga1 or under PAC treatment ( Supplementary Fig. 6 ) and degraded in response to GA by the SCF SLY1 complex [23] , these observations indicate that NF-YC function on germination inhibition requires RGL2. On the contrary, similar to rgl2 , the nf-yc mutants promote the germination of ga1 or PAC-treated seeds ( Fig. 1c,d , Supplementary Fig. 3a,b ), supporting that the repressive role of RGL2 in germination is also dependent on NF-YCs. Observation that rgl2 nf-ycT had no significant difference with rgl2 further confirmed the interdependent roles of NF-YCs and RGL2 in germination inhibition ( Fig. 3 ). 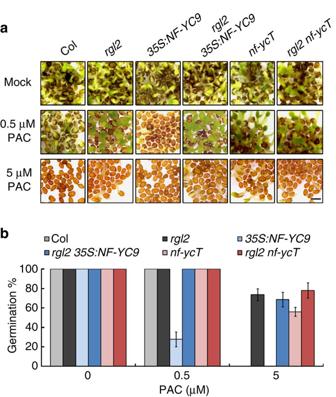Figure 3: RGL2 compromises the PAC hypersensitivity ofNF-YC9overexpression line in seed germination. (a) Germination phenotypes ofrgl2,35S:NF-YC9,rgl2 35S:NF-YC9,nf-ycT,rgl2 nf-ycTand the wild-type (Col) seeds observed at 96 HAS on 1/2 MS medium containing different concentrations of PAC. Scale bar, 1 mm. (b) Statistic analysis of germination rate in the seeds described ina. Data represent mean±s.d. of at least 100 seeds. Figure 3: RGL2 compromises the PAC hypersensitivity of NF-YC9 overexpression line in seed germination. ( a ) Germination phenotypes of rgl2 , 35S:NF-YC9 , rgl2 35S:NF-YC9 , nf-ycT , rgl2 nf-ycT and the wild-type (Col) seeds observed at 96 HAS on 1/2 MS medium containing different concentrations of PAC. Scale bar, 1 mm. ( b ) Statistic analysis of germination rate in the seeds described in a . Data represent mean±s.d. of at least 100 seeds. Full size image Further analysis demonstrated that transcriptional and protein levels of NF-YC3, NF-YC4 and NF-YC9 were rarely affected by rgl2 under mock or PAC treatment ( Supplementary Fig. 8a,c ). In turn, NF-YCs also had less effect on the transcription and protein accumulation of RGL2 ( Supplementary Fig. 8b,c,d ). These observations demonstrate that NF-YCs and RGL2 do not regulate each other in the mRNA or protein levels. Together, above data corroborate that NF-YCs and RGL2 interdependently repress seed germination via protein interactions. NF-YCs and RGL2 coregulate a set of downstream genes To understand how the NF-YC–RGL2 complex functions in repressing seed germination, a genome-wide transcriptomic analysis was carried out using germinating seeds of rgl2 , nf-ycT and the wild type (Col) with PAC and Col with mock treatment ( Supplementary Data 1 ). On the basis of the criteria of 1.5-fold cutoff for the genes with 5% false discovery rate, we first identified 1,326, 906 and 632 differentially expressed genes in Col_PAC versus Col_mock, nf-ycT _PAC versus Col_PAC, and rgl2 _PAC versus Col_PAC subsets, which are referred to as PAC-, NF-YC- and RGL2-regulated genes ( Fig. 4a , Supplementary Data 2 ). To define whether the PAC-regulated genes respond to GA, we executed a comparative analysis of the PAC-regulated genes profile with a previous microarray data in which the GA-regulated transcripts were identified from L er wild-type versus ga1-3 germinating seeds [43] , [44] , and it showed a high overlap (44.6%) between these two independent data sets despite the different ecotypes and growth conditions used ( Supplementary Data 2 ). Venn diagrams demonstrated that ∼ 70% (444/632) of RGL2-regulated genes and ∼ 41% (374/906) of NF-YC-regulated genes were also regulated by PAC mostly in an identical pattern, respectively, while ∼ 28% (174/632) of RGL2-regulated genes were similarly regulated by NF-YCs ( Supplementary Fig. 9a ), implying the high correlation of regulation between RGL2 and NF-YCs. Total 142 overlapped genes were coregulated by PAC, NF-YC and RGL2, which are considered as target genes involving in NF-YC- and RGL2-mediated seed germination ( Supplementary Data 3 ). Strikingly, most of these coregulated genes were regulated by NF-YC, RGL2 and PAC in the same direction, and only three genes (2%) were differentially regulated ( Fig. 4b , Supplementary Fig. 9b , Supplementary Data 3 ). Further gene ontology (GO) analysis revealed that these genes were primarily enriched in seed germination, response to hormone stimulus, cell wall modification, transferase activity, transport and other metabolic process ( Supplementary Data 3 ). Interestingly, in the top three GO annotations, more co-upregulated genes were involved in response to ABA (12.2%), whereas lesser of them in cell wall modification (1.2%). The co-downregulated genes were remarkably enriched in cell wall-related process (28.1%) and none of them in response to ABA (0%). By contrast, the two subsets of genes were both involved in GA-mediated seed germination (32.9 and 19.3%, respectively) ( Fig. 4c ). These data reveal that NF-YCs and RGL2 co-target a set of common genes in response to phytohormone signals, strongly supporting the role of NF-YC-RGL2 in seed germination regulation. 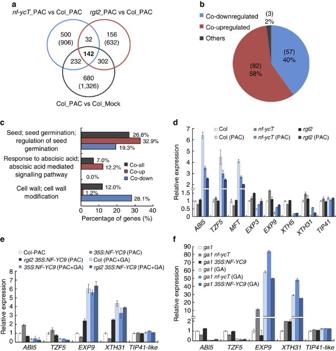Figure 4: Transcriptomic analysis of regulatory gene expression profiles by NF-YCs and RGL2 in response to GA. (a) The Venn diagram shows the coregulated genes by GA, NF-YCs and RGL2, indicated as the overlap among the differentially expressed genes innf-ycT_PAC versus Col_PAC,rgl2_PAC versus Col_PAC, and Col_PAC versus Col_Mock. (b) Percentages of the co-upregulated, the co-downregulated and the genes in the other patterns by GA, NF-YCs and RGL2. Values enclosed in parentheses indicate the numbers of genes. (c) Gene ontology analysis of the coregulated (co-all), the co-upregulated (co-up) and the co-downregulated (co-down) genes by GA, NF-YCs and RGL2. Numbers indicate the percentages of genes included in each GO category. (d) Quantitative RT–PCR analysis of the expression level of several selected cell wall-related and ABA responsive genes coregulated by GA, NF-YCs and RGL2. The wild-type (Col),rgl2andnf-ycTseeds were grown on 1/2 MS medium containing 5 μM PAC or not for 12 HAS. The relative gene expression was normalized to that ofPP2Ainternal control and then calculated by comparing the value with that in Col.TIP41-likegene was used as a negative experimental control. Data represent mean±s.d. of three biological replicates. (e) Quantitative RT–PCR analysis of the expression level of the selected coregulated genes in Col,35S:NF-YC9andrgl2 35S:NF-YC9seeds grown on 1/2 MS medium containing 5 μM PAC or 5 μM PAC plus 1 μM GA for 12 HAS. The relative gene expression was normalized to that ofPP2Ainternal control and then calculated by comparing the value with that in Col with PAC treatment (Col-PAC). Data represent mean±s.d. of three biological replicates. (f) Quantitative RT–PCR analysis of the expression level of the selected coregulated genes inga1,ga1 nf-ycTandga1 35S:NF-YC9seeds grown on 1/2 MS medium containing 1 μM GA or not for 12 HAS. The relative gene expression was normalized to that ofPP2Ainternal control and then calculated by comparing the value to that inga1. Data represent mean±s.d. of three biological replicates. Figure 4: Transcriptomic analysis of regulatory gene expression profiles by NF-YCs and RGL2 in response to GA. ( a ) The Venn diagram shows the coregulated genes by GA, NF-YCs and RGL2, indicated as the overlap among the differentially expressed genes in nf-ycT _PAC versus Col_PAC, rgl2 _PAC versus Col_PAC, and Col_PAC versus Col_Mock. ( b ) Percentages of the co-upregulated, the co-downregulated and the genes in the other patterns by GA, NF-YCs and RGL2. Values enclosed in parentheses indicate the numbers of genes. ( c ) Gene ontology analysis of the coregulated (co-all), the co-upregulated (co-up) and the co-downregulated (co-down) genes by GA, NF-YCs and RGL2. Numbers indicate the percentages of genes included in each GO category. ( d ) Quantitative RT–PCR analysis of the expression level of several selected cell wall-related and ABA responsive genes coregulated by GA, NF-YCs and RGL2. The wild-type (Col), rgl2 and nf-ycT seeds were grown on 1/2 MS medium containing 5 μM PAC or not for 12 HAS. The relative gene expression was normalized to that of PP2A internal control and then calculated by comparing the value with that in Col. TIP41-like gene was used as a negative experimental control. Data represent mean±s.d. of three biological replicates. ( e ) Quantitative RT–PCR analysis of the expression level of the selected coregulated genes in Col, 35S:NF-YC9 and rgl2 35S:NF-YC9 seeds grown on 1/2 MS medium containing 5 μM PAC or 5 μM PAC plus 1 μM GA for 12 HAS. The relative gene expression was normalized to that of PP2A internal control and then calculated by comparing the value with that in Col with PAC treatment (Col-PAC). Data represent mean±s.d. of three biological replicates. ( f ) Quantitative RT–PCR analysis of the expression level of the selected coregulated genes in ga1 , ga1 nf-ycT and ga1 35S:NF-YC9 seeds grown on 1/2 MS medium containing 1 μM GA or not for 12 HAS. The relative gene expression was normalized to that of PP2A internal control and then calculated by comparing the value to that in ga1 . Data represent mean±s.d. of three biological replicates. Full size image Further quantitative PCR with reverse transcription (RT–PCR) analysis was performed to confirm the regulation of NF-YC–RGL2 on several selected downstream genes. Consistent with the transcriptomic analysis, PAC dramatically induced the expression of ABA responsive genes ABI5 , TZF5 and MFT , and repressed that of cell wall-related genes EXP3 , EXP9 , XTH5 and XTH31 , respectively, in the wild-type germinating seeds, whereas these PAC-triggered expression changes were compromised by nf-yc and rgl2 . By contrast, these selected genes have largely comparable expression in different genetic backgrounds when grown in normal condition ( Fig. 4d ). Furthermore, the effect of GA on expression of NF-YC–RGL2 downstream was analysed in various genetic backgrounds. In the absence of GA (under PAC treatment or in ga1 background), 35S:NF-YC9 promoted the expression of ABI5 , TZF5 and repressed that of EXP9 , XTH31 , respectively. However, the transcriptional regulation effect of NF-YCs on the selected genes was significantly compromised by loss of RGL2 or GA application, similarly, the effect of RGL2 on the selected genes in ga1 was also attenuated by loss of NF-YCs or GA application ( Fig. 4e,f ). These results confirm that NF-YC–RGL2 differentially regulates two subsets of genes that are involved in ABA response and GA-mediated cell wall modification, respectively, to repress seed germination. Meanwhile, it is also intriguing how this complex functions on activation and repression of its downstream. Interestingly, the chromatin immunoprecipitation (ChIP) assay showed that, rather than the direct transcriptional repression on the cell wall-related genes, NF-YC–RGL2 module might directly target ABA responsive gene ABI5 for transcriptional activation ( Supplementary Fig. 10 ). NF-YC–RGL2 activates ABI5 by recognizing CCAAT elements The binding of NF-YC–RGL2 to chromatin provoked us to speculate whether this complex serves as a transcriptional activator to directly regulate the ABI5 gene. Because NF-Y was reported to specifically bind to the CCAAT-box in promoter of target genes [26] , [45] , we analysed the ABI5 genomic DNA and chose 12 fragments (P1 to P12), which covered all six CCAAT-boxes of the ABI5 region, for next examination ( Fig. 5a ). ChIP analyses of PAC-treated nf-yc9 pNF-YC9:NF-YC9-3FLAG and rgl2 pRGL2:RGL2-6HA seeds revealed that both NF-YC9 and RGL2 were associated with the genomic region near the adjacent fragments P7 and P8 with the highest enrichments ( Fig. 5a ). ChIP–reChIP analysis further verified that NF-YC9 and RGL2 co-localized to the same region of ABI5 ( Fig. 5a ). Since P7 and P8 fragments contained two CCAAT elements (designated as CCAAT-2 and CCAAT-3, respectively), to examine whether these elements are involved in the NF-YC–RGL2 regulation on ABI5 expression, we performed transient expression assays using ∼ 1.8 kb fragment of native or various mutated ABI5 promoters fused to the β-glucuronidase ( GUS ) reporter gene. The effector constructs of 35S:NF-YC9 and 35S:RGL2 were individually or together transfected with reporters into Arabidopsis mesophyll protoplasts ( Fig. 5b ). Addition of RGL2 or NF-YC9 activated the expression of ABI5 . Notably, in comparison with that expressing RGL2 alone, the higher GUS activity was detected when co-expressing NF-YC9 and RGL2 ( Fig. 5b ). However, when site-specific mutations (CCAAT to ACATA) were introduced into the CCAAT elements in ABI5 promoter, the expression of ABI5 was strikingly impaired by disruption of the CCAAT-2 or CCAAT-3 (Mut2 or Mut3) but not by Mut1 or Mut4, either each or both NF-YC9 and RGL2 existed ( Fig. 5b ). These results indicate that the CCAAT elements located at P7 and P8 are essential for NF-YC–RGL2-mediated activation of ABI5 . In addition, other DELLA proteins also contribute to ABI5 expression activation together with NF-YC9 in a variable extent ( Supplementary Fig. 11 ). Since the different circumstances between cells of protoplasts and germinating seeds, the biological roles of these DELLAs on ABI5 in plants still need to be further determinated. 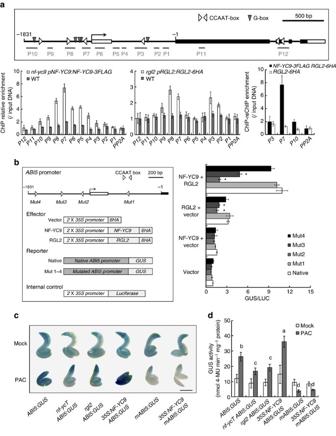Figure 5: NF-YCs and RGL2 synergistically regulateABI5expression by binding to theABI5promoter. (a) ChIP and ChIP-reChIP analyses of NF-YC9 and RGL2 binding to CCAAT-box containing region inABI5genes upon precipitation with anti-FLAG or/and anti-HA antibodies in the WT (wild-type, Col-0),nf-yc9 pNF-YC9:NF-Y9-3FLAG,rgl2 pRGL2:RGL2-6HA(RGL2-6HA) andrgl2 nf-yc9 pNF-YC9:NF-YC9-3FLAG pRGL2:RGL2-6HA(NF-YC9-3FLAG RGL2-6HA) lines. The seeds were grown on 1/2 MS medium containing 5 μM PAC for 12 HAS and harvested for further test. Relative enrichment fold was calculated by normalizing the amount of a target DNA fragment against that of a genomic fragment of a reference geneTUB8, and then against the respective input DNA samples. The enrichment of aPP2Agenomic fragment was used as the negative control (the same below). Data represent mean±s.d. of biological triplicates. (b) Transient expression assays ofABI5promoter activity modulated by NF-YC9 and RGL2 inArabidopsismesophyll protoplasts. Various constructs used in transient expression assays are shown in the left panel. EitherABI5:GUS(Native) or fourmABI5:GUS(Mut1∼4) were co-transformed with effectors or the empty vector (Vector) into Col mesophyll protoplasts. Relative GUS activity (GUS/Luciferase) that indicates the level ofABI5expression activated by various effectors is shown in the right panel. Data represent mean±s.d. of three biological replicates. Asterisks indicate significant changes of samples when compared with the relevant native sample (Student’st-test,P<0.05). (c) Representative GUS staining of mock (upper panel) and PAC treated (lower panel) seeds harbouringABI5:GUSor its mutated version in various genetic backgrounds. The seeds were grown on 1/2 MS either containing 5 μM PAC or mock for 48 HAS. Scale bar, 0.5 mm. (d) Quantitative analysis of GUS activity in the native and mutatedABI5:GUSseeds shown inc. Data represent mean±s.d. from at least 100 seeds of each genotype. Statistically significant differences are indicated by different lower-case letters (Student’st-test,P<0.05). Figure 5: NF-YCs and RGL2 synergistically regulate ABI5 expression by binding to the ABI5 promoter. ( a ) ChIP and ChIP-reChIP analyses of NF-YC9 and RGL2 binding to CCAAT-box containing region in ABI5 genes upon precipitation with anti-FLAG or/and anti-HA antibodies in the WT (wild-type, Col-0), nf-yc9 pNF-YC9:NF-Y9-3FLAG , rgl2 pRGL2:RGL2-6HA ( RGL2-6HA ) and rgl2 nf-yc9 pNF-YC9:NF-YC9-3FLAG pRGL2:RGL2-6HA ( NF-YC9-3FLAG RGL2-6HA ) lines. The seeds were grown on 1/2 MS medium containing 5 μM PAC for 12 HAS and harvested for further test. Relative enrichment fold was calculated by normalizing the amount of a target DNA fragment against that of a genomic fragment of a reference gene TUB8 , and then against the respective input DNA samples. The enrichment of a PP2A genomic fragment was used as the negative control (the same below). Data represent mean±s.d. of biological triplicates. ( b ) Transient expression assays of ABI5 promoter activity modulated by NF-YC9 and RGL2 in Arabidopsis mesophyll protoplasts. Various constructs used in transient expression assays are shown in the left panel. Either ABI5:GUS (Native) or four mABI5:GUS (Mut1 ∼ 4) were co-transformed with effectors or the empty vector (Vector) into Col mesophyll protoplasts. Relative GUS activity (GUS/Luciferase) that indicates the level of ABI5 expression activated by various effectors is shown in the right panel. Data represent mean±s.d. of three biological replicates. Asterisks indicate significant changes of samples when compared with the relevant native sample (Student’s t -test, P <0.05). ( c ) Representative GUS staining of mock (upper panel) and PAC treated (lower panel) seeds harbouring ABI5:GUS or its mutated version in various genetic backgrounds. The seeds were grown on 1/2 MS either containing 5 μM PAC or mock for 48 HAS. Scale bar, 0.5 mm. ( d ) Quantitative analysis of GUS activity in the native and mutated ABI5:GUS seeds shown in c . Data represent mean±s.d. from at least 100 seeds of each genotype. Statistically significant differences are indicated by different lower-case letters (Student’s t -test, P <0.05). Full size image Because no DNA binding domain is identified in DELLA proteins, to make clear how RGL2 and NF-YC9 recognize ABI5 promoter, we performed protein–DNA affinity pull-down assay in which a heterotrimeric NF-Y, composed of NF-YC9 and two NF-Y subunits core domains from yeast (NF-YA core and NF-YB core), was used for CCAAT element binding as previously reported [46] . Interestingly, RGL2 indirectly associated with the ABI5 promoter fragment DNA containing CCAAT-2/3 ( ABI5-2,3 ), but not with the mutated ABI5-2,3 or ABI5 promoter fragment containing CCAAT-4 ( ABI5-4 ), via interacting with NF-YA core/NF-YB core/NF-YC9 complex ( Supplementary Fig. 12 ). However, the DNA affinity of RGL2-NF-YC9 was not detected in vitro ( Supplementary Fig. 12 ), which is consistent with the previous reports that NF-YC subunit has no DNA binding ability [26] . These results indicate that RGL2, not itself, but via NF-Y complex, recognizes ABI5 promoter region. To further examine whether NF-YC–RGL2 regulates ABI5 expression through the CCAAT elements during seed germination, we created ABI5:GUS transgenic plants and two mutated lines containing the Mut2 or Mut3 version of CCAAT elements. Among 11 transformants harbouring Mut2 ( mABI5:GUS ) with PAC treatment, 9 displayed significantly reduced GUS staining in comparison with ABI5:GUS seeds (data not shown). The similar results were observed in the transgenic lines harbouring Mut3 ( m3-ABI5:GUS ) ( Supplementary Fig. 13a,b ). These observations verified that CCAAT-2 and CCAAT-3 are critical for GA-mediated ABI5 expression during seed germination. Furthermore, with PAC treatment, the staining of ABI5:GUS seeds was remarkably weaker in both nf-ycT and rgl2 than that in the wild-type background, whereas there was no significant difference of GUS staining among these germinating seeds with mock treatment ( Fig. 5c,d ). As expected, ABI5:GUS but not mABI5:GUS seeds displayed an increased GUS staining in 35S:NF-YC9 compared with the wild-type background ( Fig. 5c,d ). Thus, these findings strongly support the idea that NF-YC–RGL2 module activates ABI5 expression via binding to the specific CCAAT elements. It was noted that, although PAC resulted in increased GUS staining in the ABI5:GUS seeds, but it had an opposite effect on the mABI5:GUS seeds probably owing to other unknown regulations caused by the disruption of CCAAT element. ABI5 is epistatic to NF-YCs and RGL2 Because NF-YCs and RGL2 interact to directly regulate ABI5 expression, we wondered whether NF-YCs and RGL2 are cooperative and interdependent on such transcriptional regulation. ChIP analyses of rgl2 nf-yc9 pNF-YC9:NF-YC9-3FLAG and nf-ycT rgl2 pRGL2:RGL2-6HA showed that the absence of RGL2 significantly impaired the affinity of NF-YC9 to P7/8 fragments in ABI5 promoter. In turn, binding of RGL2 to the same locus was attenuated by nf-ycT ( Fig. 6a ). Furthermore, GA application also weakened the DNA binding of NF-YC9 in PAC-treated seeds ( Supplementary Fig. 14 ). The results suggest that NF-YCs and RGL2 cooperatively bind to the CCAAT elements to regulate ABI5 transcription. 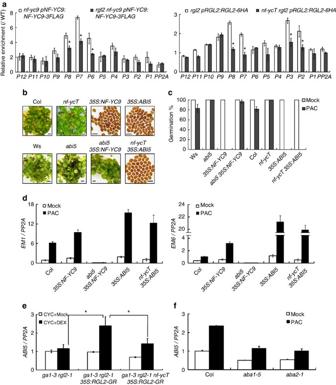Figure 6: ABI5 is required for NF-YC–RGL2-mediated seed germination. (a) ChIP analysis of NF-YC9 or RGL2 binding to CCAAT-box containing regions ofABI5promoter upon precipitation with anti-FLAG or anti-HA antibodies in seeds under various genetic backgrounds. The seeds were grown on 1/2 MS medium containing 5 μM PAC for 12 HAS and harvested for ChIP assay. Data represent mean±s.d. of triplicates. Asterisks indicate significant changes in ChIP-enrichment fold between crossed lines and relevant parent lines (Student’st-test,P<0.05). (b) Germination phenotypes of seeds in various genetic backgrounds observed at 120 HAS on 1/2 MS medium containing 1 μM PAC. (c) Statistic analysis of germination rate in the seeds described inb. Germination rate in all the seeds with mock treatment is 100%. Data represent mean±s.d. of at least 100 seeds. Scale bar, 1 mm. (d) Quantitative RT–PCR analysis ofEM1andEM6expression in seeds in various genetic backgrounds grown on 1/2 MS medium containing 5 μM PAC or not for 12 HAS. (e) Quantitative RT–PCR analysis ofABI5expression inga1-3 rgl2-1,ga1-3 rgl2-1 35S:RGL2-GRandga1-3 rgl2-1 nf-ycT 35S:RGL2-GRseeds grown on 1/2 MS medium containing 10 μM cyclohexanone (CYC) or 10 μM CYC plus 10 μM dexamethasone (DEX) for 4 h. Data represent mean±s.d. of three replicates. Asterisks indicate significant changes between the selected samples (Student’st-test,P<0.05). (f) Quantitative RT–PCR analysis ofABI5expression inaba1-5,aba2-1and the wild-type seeds grown on 1/2 MS medium containing 5 μM PAC or not for 12 HAS. Data represent mean±s.d. of three replicates. Figure 6: ABI5 is required for NF-YC–RGL2-mediated seed germination. ( a ) ChIP analysis of NF-YC9 or RGL2 binding to CCAAT-box containing regions of ABI5 promoter upon precipitation with anti-FLAG or anti-HA antibodies in seeds under various genetic backgrounds. The seeds were grown on 1/2 MS medium containing 5 μM PAC for 12 HAS and harvested for ChIP assay. Data represent mean±s.d. of triplicates. Asterisks indicate significant changes in ChIP-enrichment fold between crossed lines and relevant parent lines (Student’s t -test, P <0.05). ( b ) Germination phenotypes of seeds in various genetic backgrounds observed at 120 HAS on 1/2 MS medium containing 1 μM PAC. ( c ) Statistic analysis of germination rate in the seeds described in b . Germination rate in all the seeds with mock treatment is 100%. Data represent mean±s.d. of at least 100 seeds. Scale bar, 1 mm. ( d ) Quantitative RT–PCR analysis of EM1 and EM6 expression in seeds in various genetic backgrounds grown on 1/2 MS medium containing 5 μM PAC or not for 12 HAS. ( e ) Quantitative RT–PCR analysis of ABI5 expression in ga1-3 rgl2-1 , ga1-3 rgl2-1 35S:RGL2-GR and ga1-3 rgl2-1 nf-ycT 35S:RGL2-GR seeds grown on 1/2 MS medium containing 10 μM cyclohexanone (CYC) or 10 μM CYC plus 10 μM dexamethasone (DEX) for 4 h. Data represent mean±s.d. of three replicates. Asterisks indicate significant changes between the selected samples (Student’s t -test, P <0.05). ( f ) Quantitative RT–PCR analysis of ABI5 expression in aba1-5 , aba2-1 and the wild-type seeds grown on 1/2 MS medium containing 5 μM PAC or not for 12 HAS. Data represent mean±s.d. of three replicates. Full size image ABI5 functions as the central ABA signalling component to repress seed germination, which is epistatic to RGL2 (ref. 23 ). To investigate the genetic role of NF-YCs in ABI5-mediated inhibition of seed germination, we created abi5 35S:NF-YC9 combinatorial line and found that loss of ABI5 strikingly suppressed the hypersensitivity of 35S:NF-YC9 to PAC in germinating seeds ( Fig. 6b,c ). Consistent with this, the expression of two ABI5 target genes EM1 and EM6 was decreased in abi5 35S:NF-YC9 compared with 35S:NF-YC9 seeds ( Fig. 6d ). In turn, overexpression of ABI5 remarkably rescued the PAC-reduced sensitivity of nf-ycT ( Fig. 6b,c ), and EM1 and EM6 genes expressed at comparable levels in 35S:ABI5 and nf-ycT 35S:ABI5 seeds ( Fig. 6d ). These results, together with previous report [23] , suggest that ABI5 act epistatic to NF-YCs and RGL2 during seed germination. We next examined the ABI5 expression in response to immediate RGL2 activity using a steroid-inducible RGL2 (RGL2-GR) in ga1-3 rgl2-1 background. In contrast to no change in ga1-3 rgl2-1 , ABI5 expression was rapidly induced by dexamethasone combined with cycloheximide in ga1-3 rgl2-1 35S:RGL2-GR without de novo protein synthesis, whereas it was compromised in ga1-3 rgl2-1 nf-ycT 35S:RGL2-GR ( Fig. 6e ), providing a further molecular evidence to support genetic relationship between NF-YC–RGL2 and ABI5 . Previous studies showed that GA promotes seed germination by triggering RGL2 degradation, and RGL2 indirectly regulates ABI5 expression through stimulating ABA biosynthesis, thus inhibiting germination [23] , [47] , [48] . Here, our observations support a direct regulation of RGL2 on ABI5 . To determine whether such regulation is ABA dependent or not, we examined the expression of ABI5 in ABA synthesis defective mutants aba1-5 and aba2-1 . Interestingly, the ABI5 expression was still induced, even though with lesser elevated extent than the wild-type, in PAC-treated aba1 and aba2 seeds compared with mock-treated ( Fig. 6f ), implying ABI5 might be regulated by GA or RGL2 regardless of ABA biosynthesis. NF-YC–RGL2 functions in ABA-mediated germination inhibition Germination process contains the rupture of the testa before the endosperm rupture. ABA suppresses seed germination mainly through inhibition of endosperm rupture rather than that of testa rupture, whereas RGL2 accumulation prevents both testa and endosperm rupture under GA deficiency [10] , [23] . We here investigated the detailed role of NF-YCs in testa and endosperm rupture. Under normal condition, the germination rates of all examined seeds were 100% at 120 HAS ( Fig. 7a,b ). In the presence of ABA, compared with the wild-type, nf-ycT , rgl2 and abi5 showed higher testa and endosperm rupture rates, but the 35S:NF-YC9 seeds had the lower rate on those ( Fig. 7a,b ). Furthermore, 35S:ABI5 dramatically attenuated or abolished the ABA insensitivity of nf-ycT and rgl2 , while abi5 35S:NF-YC9 still remained high testa and endosperm rupture rates as abi5 . In addition, loss of ABI5 function also significantly rescued non-germinating phenotype of ga1 under either ABA or mock treatment ( Fig. 7a,b ). The results indicate that, similar to RGL2, NF-YCs repress both testa and endosperm rupture via ABI5 in ABA-mediated seed germination. 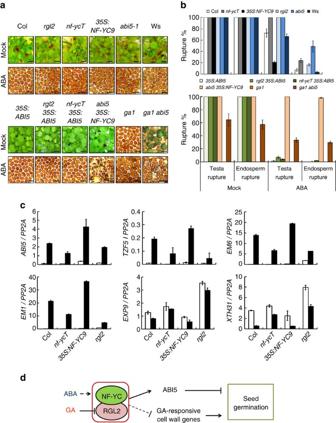Figure 7: NF-YCs and RGL2 are involved in the ABA-mediated inhibition of germination. (a) Germination phenotypes ofrgl2,nf-ycT,abi5,35S:NF-YC9,35S:ABI5, the wild-type (Col and Ws) seeds and their combinatorial lines observed at 120 HAS on 1/2 MS medium containing 2 μM ABA or not (mock). Scale bar, 1 mm (b) Statistic analysis of the testa and endosperm rupture rate in germinating seeds described ina. Data represent mean±s.d. of at least 100 seeds. (c) Quantitative RT–PCR analysis of several representative genes expression innf-ycT,35S:NF-YC9,rgl2and the wild-type seeds grown on 1/2 MS medium containing 2 μM ABA or not for 12 HAS. Data represent mean±s.d. of three replicates. (d) A model of NF-YC-RGL2-mediated seed germination by integrating GA and ABA signalling. Solid lines indicate the direct or definite regulation; dotted lines indicate the indirect or undetermined regulation. Figure 7: NF-YCs and RGL2 are involved in the ABA-mediated inhibition of germination. ( a ) Germination phenotypes of rgl2 , nf-ycT , abi5 , 35S:NF-YC9 , 35S:ABI5 , the wild-type (Col and Ws) seeds and their combinatorial lines observed at 120 HAS on 1/2 MS medium containing 2 μM ABA or not (mock). Scale bar, 1 mm ( b ) Statistic analysis of the testa and endosperm rupture rate in germinating seeds described in a . Data represent mean±s.d. of at least 100 seeds. ( c ) Quantitative RT–PCR analysis of several representative genes expression in nf-ycT , 35S:NF-YC9 , rgl2 and the wild-type seeds grown on 1/2 MS medium containing 2 μM ABA or not for 12 HAS. Data represent mean±s.d. of three replicates. ( d ) A model of NF-YC-RGL2-mediated seed germination by integrating GA and ABA signalling. Solid lines indicate the direct or definite regulation; dotted lines indicate the indirect or undetermined regulation. Full size image To further determine the regulatory effect of NF-YC–RGL2 module on ABA-mediated seed germination, we examined the transcriptional level of several representative NF-YC–RGL2 coregulated genes in different seeds under ABA treatment. As expected, all selected genes in the ABA-treated seeds of nf-ycT , rgl2 and 35S:NF-YC9 were expressed in similar regulatory patterns with those under PAC treatment ( Fig. 7c , Fig. 4d,e , Supplementary Fig. 15 ). These results collectively support the conclusion that NF-YC–RGL2 module integrates ABA and GA signalling to regulate seed germination. Numerous genetic and physiological studies have documented the antagonistic roles of GA and ABA, which are essential for seeds to determine whether germination starts or not. DELLA protein RGL2, the main GA signalling repressor in germination, serves as a central modulator in such process [16] , [19] , [20] . GA-triggered degradation of DELLAs by ubiquitin–proteasome pathway or repression of DELLAs by nonproteolytic GA signalling promotes normal seeds germination [18] , [47] , [48] . Here, we demonstrate that three Arabidopsis NF-YC homologues interact with RGL2 protein to interdependently regulate a set of genes involved in GA-related cell wall modification and ABA response, especially ABI5 , the gene encoding a core component of ABA signalling, thus, control seed germination ( Fig. 7d ). In imbibing seeds, bioactive GA is produced to decrease RGL2 accumulation, thus mediating ABI5-regulated ABA signalling and accelerating germination process. These results illustrate a hypothetic regulatory model of phytohormones crosstalk and reveal a direct molecular link of NF-YC–RGL2–ABI5 that integrates GA and ABA signalling to precisely regulate seed germination, providing new insights into understanding on how DELLAs mediate the antagonism between GA and ABA via a direct signalling modulation. Consistent with antagonistic roles of GA and ABA in germination, GA synthesis promptly ascends, while ABA content decreases, in imbibed seeds [4] , [5] . Furthermore, it has been showed that the ABA synthesis deficient mutant aba2 seeds have higher endogenous GA levels [49] , and in turn, the ABA synthesis is enhanced in the GA-deficient mutant ga1-3 (ref. 41 ). ABI5 plays a vital role in repressing the germination of nondormant seeds, and its transcriptional expression and protein activity respond to changes in ABA and GA levels. The studies have suggested that RGL2 stimulates endogenous ABA synthesis probably via XERICO, a RING-H2 factor promoting ABA accumulation in an unknown manner, thus activating ABI5 expression [23] , [25] . However, we here reveal a direct regulation of RGL2 in ABI5 transcription through interacting with NF-YCs. This is further corroborated by the observations that PAC induces the expression of ABI5 even in the absence of ABA ( aba1 and aba2 background), and immediate upregulation of ABI5 by the inducible RGL2 does not need de novo protein synthesis ( Fig. 6e,f ), suggesting that RGL2 is able to directly regulate ABI5 gene in an ABA-independent manner. It is also noteworthy that the PAC-induced ABI5 expressions are lower in aba1-5 and aba2-1 than that in the wild-type ( Fig. 6f ). This is probably due to the decreased mRNA and protein level of RGL2 in ABA-deficient mutants [23] . Considering that the stability and activity of ABI5 protein are mostly dependent on ABA levels [23] , and changes of ABA or ABI5 level affect the sensitivity of germinating seeds to PAC [13] ( Fig. 6b,c ), ABA may act as an important modulator in fine-tuning the regulation of NF-YC–RGL2–ABI5 hierarchical cascade on seed germination. The transcriptomic analysis reveals that the RGL2–NF-YC modulates two subsets of different downstreams including ABA responsive and cell wall-related genes in germination. It is noteworthy that in addition to the main effect in blocking GA biosynthesis, PAC used in this analysis might cause an undesirable increase of ABA levels by interfering in ABA catabolism [39] . A comparative analysis of the PAC-regulated genes with a previously identified GA-regulated expression profile [43] exhibited high overlapping between these two independent data sets, together with the expression analysis of the selected genes, supporting that the majority of PAC-regulated genes is responsive to GA. TZF4/SOM and TZF5 , encoding two functional CCCH zinc finger proteins presented in co-upregulated genes profile, repress seed germination by controlling GA and ABA responsive genes expression [50] , [51] . MFT, another co-upregulated gene product, is involved in seed germination regulation through a negative feedback loop modulating ABA signalling pathway [52] . We hence speculate that NF-YC–RGL2 might act as a key node to induce ABA responsive gene expression and to repress GA-related cell wall genes expression partially via activating a number of transcriptional regulators such as ABI5, TZF4/SOM, TZF5 and MFT ( Fig. 4 , Supplementary Data 3 ). The α-amylase gene encodes starch hydrolase and acts as a classic downstream gene under the antagonistic regulation between GA and ABA in cereal seeds germination [53] . In the barley aleurone, GAMYB , encoding a well-known GA-related transcription factor that induces the expression of α-amylase gene, is promoted by GA-triggered degradation of DELLA protein SLN1 and repressed by the ABA-induced protein kinase PKABA1 (refs 53 , 54 ). Our transcriptomic analysis and ChIP assays did not detect the direct regulation by DELLA-NF-YC module in these genes. How α-amylase encoding AtAMYs and GAMYB are regulated by GA and ABA signalling in Arabidopsis germinating seeds, and whether the DELLA-NF-YC module works in cereal plants, remain to be investigated in future. As transcriptional regulators, DELLA proteins exert their function by interfering with other transcription factors rather than directly binding to their target genes [55] , [56] , [57] . However, the increasing evidences revealed that DELLAs also likely activate or repress downstream genes expression through directly targeting their promoters [25] , [44] , [58] , [59] , [60] . Our observation of ABI5 activation by NF-YC–RGL2 further confirm this, supporting the dual role of DELLA presented in ‘the targeting model’ and ‘relief of repression model’ as described previously [57] , [58] . NF-YC associates with NF-YA and NF-YB subunits by the HFD domain for recognition of CCAAT element in eukaryotes [26] . Recent studies also showed the CCAAT binding of plant NF-Y heterotrimer by several combinations of NF-Y subunits in vitro or in vivo [31] , [33] , [45] , [61] . In addition, canonical CCAAT boxes were identified as important repressive transcription regulatory elements in promoters of rice GAMYB and RPBF , the genes involved in GA regulation of expression during germination of rice seeds [62] . In our observations, RGL2 interacts with the non-HFD C terminus of NF-YCs to co-locate at the CCAAT elements in ABI5 , implying that specific NF-Y complexes might function with RGL2 together in control of seed germination. Further protein–DNA affinity pull-down assay confirms the direct binding of NF-Y–RGL2 to the ABI5 promoter, and that RGL2 indirectly recognizes CCAAT elements via NF-Y complex. Notably, there are three G-box elements (CACGTG) contained between the two functional CCAAT sites ( Fig. 5a ). These G-box are bound by ABI5 itself in yeast [63] . Hence, it raises concern that RGL2 and NF-YCs probably play a role in mediating ABI5 self-regulation. Previous studies reported that NF-YC3, NF-YC4 and NF-YC9 redundantly function in cooperation with GA response to promote flowering, which is in turn repressed by DELLAs via protein interaction [30] , [36] . However, our results indicate that these NF-YCs together with DELLAs oppose GA response for seed germination inhibition. Because NF-Y functions as the important regulators that widely mediate plant development and environmental responses [27] , this opposite role of NF-YCs between germination and flowering processes might be caused by the spatio-temporal regulation of NF-Y complexes consisted of diverse NF-YA/B/C on different sets of target genes in various development stages. In addition, DELLAs also have distinct functions other than overlapping roles in plant development. For instance, RGL2 functions as the central repressor in GA-mediated and light-dependent germination, while RGA and GAI synergistically repress plant vegetative growth [15] , [20] , [23] . Hence, it is worthy to identify different combinations of DELLA-NF-Y(C) that function in different biological processes, such as cell expansion, tissue development and stress responses. Taken together, we reveal a key regulatory module NF-YC–RGL2 by which GA directly intervenes in ABA signalling, and thus regulates seed germination. These findings provide novel insights into mechanism of antagonism between GA and ABA during plant development. Plant materials and growth conditions All Arabidopsis plants used in this study are in Col background except for ga1-3 rgl2-1 and ga1-3 rgl2-1 35S:RGL2-GR in L er background, and abi5-1 in Ws background. The nf-yc3-2 (GK-051E10), nf-yc4-1 (SALK_032163), nf-yc9-1 (SALK_058903), ga1 (SALK_109115), rgl2 (SALK_124231) and rga-28 (SALK_089146) seeds were obtained from the ‘The Arabidopsis Information Resource (TAIR, http://www.arabidopsis.org/ ). Transgenic lines of 35S:NF-YC3-6HA , 35S:NF-YC9-6HA and nf-yc9-1 pNF-Y9:NF-YC9-3FLAG and the mutants of aba1-5 and aba2-1 (refs 13 , 36 ). Each transgenic line used to compare under different genetic backgrounds in this study is the same line which was introduced into various mutants by crossing. The seeds used for germination comparison were harvested in the same batch of plants grown at 22 °C under long days (16 h light/8 h dark). Dry seeds were obtained and stored in a dry condition (25% humidity, 25 °C) for at least 4 weeks of after-ripening before performing the germination test. Genes referenced in this article can be found in the Arabidopsis Genome Initiative database under the following accession numbers: NF-YC3 (AT1G54830), NF-YC4 (AT5G63470), NF-YC9 (AT1G08970), RGL2 (AT3G03450), RGA (AT2G01570), RGL1 (AT1G66350), GAI (AT1G14920), RGL3 (AT5G17490), ABI5 (AT2G36270), TZF5 (AT5G44260), MFT (AT1G18100), EM1 (AT3G51810), EM6 (AT2G40170), XTH5 (AT5G13870), XTH31 (AT3G44990), EXP3 (AT2G37640), EXP9 (AT5G02260), PP2A (AT1G13320), TIP41-like (AT4G34270) and TUB8 (AT5G23860). Seed germination assay The after-ripened seeds were sterilized and washed with 75% (v/v) ethanol with 0.5% (v/v) Triton X-100 (Sigma-Aldrich) for 1 min, and washed twice with absolute ethanol, then were plated on sterile filter paper for air drying. Subsequently, the sterilized seeds were sown on half-strength MS medium (0.025% MES, pH 5.7) containing 0.8% (w/v) Bacto Agar (Difco/BD) supplemented with 0.01% (w/v) ethanol (Mock), PAC (Sigma-Aldrich), ABA (Sigma-Aldrich), GA 3 (Sigma-Aldrich) or DEX (Sigma-Aldrich) upon the experiment requirement. All the plates were kept at 4 °C in darkness for 3 days for stratification and then transferred to an illumination incubator at 22 °C with 16 h light/8 h dark condition for further analysis. At least 100 seeds for each genotype were used in three biological replicates. The germination event was defined as the first sign of radicle emergence and recorded at different time points until 120 h of incubation. Plasmid construction and plant transformation For the pRGL2:RGL2-6HA construct, an ∼ 3.7 kb genomic fragment of RGL2 without stop codon was amplified and cloned into the pHY105-6HA binary vector [57] . To construct 35S:RGL2-6HA , the CDS encoding RGL2 was amplified and cloned into pGreen-35S-6HA. For the ABI5:GUS construct, ∼ 1.8 kb promoter of ABI5 was cloned into the pHY107 vector harbouring the GUS reporter [57] . The primers used for plasmid construction are listed in Supplementary Table 1 . Transgenic plants harbouring pNF-YC9:NF-YC9-3FLAG were selected on 1/2 MS medium supplemented with gentamicin, while other transgenic plants were selected by basta. Yeast two-hybrid assay The coding regions of NF-YC3 , NF-YC4 , NF-YC9 , RGL2 and RGA or truncated versions of NF-YC9 and RGL2 were amplified and cloned into pGBKT7 and pGADT7 (Clontech), respectively. The primers used are listed in Supplementary Table 1 . Yeast two-hybrid assays were performed using the Yeastmaker Yeast Transformation System 2 (Clontech). Yeast AH109 cells were co-transformed with the specific bait and prey constructs. All yeast transformants were grown on SD/-Trp/-Leu or SD/-Trp/-Leu/-His/-Ade medium for selection or interaction test. BiFC analysis The coding regions of NF-YC9 and RGL2 were cloned into the serial pGreen binary vectors containing C- or N-terminal fusions of EYFP to generate 35S:NF-YC9-nEYFP and 35S:RGL2-cEYFP . Plasmids were co-transformed into Arabidopsis mesophyll protoplasts by the PEG-mediated transient transformation [64] , and then cultured for 12 h and observed for BiFC analysis using a confocal laser scanning microscope (LSM 510 META, Zeiss). In vitro pull-down assay The coding regions of NF-YC3 , NF-YC4 , NF-YC9 and RGL2 were cloned into the pQE30 (QIAGEN) and pGEX-4T-1 (Pharmacia) vectors to produce His-NF-YC3, His-NF-YC4, His-NF-YC9 and GST-RGL2 proteins, respectively. Primers used for constructions are listed in Supplementary Table 1 . GST and His fusion recombinant proteins were induced by IPTG and expressed in E. coli Rosetta (DE3, Novagen). The soluble His and GST fusion proteins were purified using Ni-NTA agarose beads (30210, QIAGEN) or Glutathione Sepharose Beads (17-0756-01, Amersham Biosciences) according to the manufacturers’ instruction. For pull-down assays, 2 μg of His-NF-YCs were incubated in the binding buffer (50 mM Tris-HCl, pH 8.0, 100 mM NaCl and 1 mM EDTA) with immobilized GST or GST fusion protein at 4 °C for 2 h. After washing with binding buffer, proteins retained on the beads were subsequently resolved by SDS loading buffer and then run SDS–PAGE to detect with anti-His (AbM59012-18-PU, BGI) at a dilution of 1:5,000 or anti-GST antibody (AB101-02, Tiangen) at a dilution of 1:2,000. Uncropped scans of western blot results are shown in Supplementary Fig. 16 . Co-immunoprecipitation assay The 5 μM PAC-treated nf-yc9 rgl2 pNF-YC9:NF-YC9-3FLAG pRGL2:RGL2-6HA seeds were kept under light for 12 h. Total proteins were extracted with extraction buffer (50 mM Hepes, pH 7.5, 150 mM NaCl, 5 mM DTT, 1% Triton X-100), and were incubated with Protein G PLUS/Protein A-Agarose Suspension (IP10, CALBIOCHEN) plus either anti-FLAG antibody (F3165, Sigma) or preimmune serum (IgG) in the co-immunoprecipitation buffer (50 mM Hepes, pH 7.5, 150 mM KCl, 10 μM ZnSO 4 , 5 mM MgCl 2 , 1% Triton X-100) at 4 °C for 2 h. After being washed by co-immunoprecipitation buffer three times, the proteins bound to beads were resolved by SDS–PAGE and detected by anti-FLAG (F3165, Sigma) at a dilution of 1:10,000 or anti-HA antibody (sc-7392, Santa Cruz) at a dilution of 1:2,000. Uncropped scans of western blot results are shown in Supplementary Fig. 16 . RNA-seq analysis The after-ripened seeds (4 weeks) harvested in a same batch were grown on half-strength MS medium (0.025% MES, pH 5.7) containing 5 μM PAC under light for 12 h. Total RNA was extracted from harvested seeds by Plant RNA Kit (R6827, Omega) and sent to BGI for RNA-seq analysis. The used RNA samples have been strictly detected upon the RNA sequencing standard and the libraries constructed using Ultra RNA sample preparation kit (Illumina) reached high quality before RNA-sequencing. Sequencing was performed using an Illumina HiSeq2000 according to the standard protocol. Total RNA-Seq reads were mapped to the Arabidopsis TAIR10 genome. The differentially expressed genes were identified by the program Cuffdiff with the criteria set as fold change >1.5 and FDR-adjusted P values <0.05. Three valid biological replicates were used for the transcriptomic analysis. The gene expression patterns were graphically represented in a heat map by cluster analysis tool in Heml software [65] . GO analysis was performed by the GO Annotation of TAIR [66] . Gene expression analysis The treatment of seeds was performed upon various experiments. Total RNA was extracted using the Plant RNA Kit (Omega) and reverse transcribed using the M-MLV reverse transcriptase (Promega). Quantitative RT–PCR was performed in triplicates on Roche LightCycler480 real-time system with the SYBR Premix ExTaq Mix (DRR041A, TaKaRa) following the manufacturer’s instruction. The relative expression level was normalized to that of PP2A internal control. The primers used for gene expression analysis are listed in Supplementary Table 1 . ChIP and ChIP–reChIP assays To perform ChIP assays, the nf-yc9 pNF-YC9:NF-YC9-3FLAG, rgl2 pRGL2:RGL2-6HA and the Col wild-type seeds were incubated with mock, 5 μM PAC or 5 μM PAC plus 1 μM GA for 12 h and harvested for fixation. Chromatins were isolated and sonicated to generate DNA fragment with an average size around 250–500 bp. The solubilized chromatins were immunoprecipitated by Protein G PLUS agarose (16–201, Millipore) with anti-FLAG (F3165, Sigma) and anti-HA (sc-7392x, Santa Cruz), and the co-immunoprecipitated DNA was recovered and analysed by quantitative PCR (qPCR) with SYBR Premix ExTaq Mix (DRR041A, TaKaRa Bio). For ChIP–reChIP assays, nf-yc9 rgl2 pNF-YC9:NF-YC9-3FLAG pRGL2:RGL2-6HA and pRGL2:RGL2-6HA seeds were incubated under 5 μM PAC for 12 h and harvested for fixation. The sonicated chromatins were immunoprecipitated by anti-HA agarose conjugate (the first ChIP), and then washed by the ChIP buffer and eluted with 10 mM dithiothreitol (DTT). The eluted chromatins were diluted 20-fold with dilution buffer (1% Triton X-100, 2 mM EDTA, 20 mM Tris-HCl at pH 8.1, 150 mM NaCl) and immunoprecipitated again by anti-FLAG (the second ChIP). The recovered DNA was purified and quantified by qPCR. Relative enrichment fold was calculated by normalizing the amount of a target DNA fragment against that of a genomic fragment of a reference gene TUB8 , and then against the respective input DNA samples. The enrichment of a PP2A genomic fragment was used as the negative control. The primers used are listed in Supplementary Table 1 . Transient expression assay To generate the ABI5:GUS reporter construct, ∼ 1.8 kb ABI5 promoter was cloned into HY107 containing GUS gene [36] . The mABI5:GUS constructs carrying mutated CCAAT elements were generated by overlapping PCR reaction from the ABI5:GUS construct. The 35S:NF-YC9-6HA and various DELLA constructs were used as effectors, and a construct containing the firefly luciferase driven by 35S promoter in pGreen-35S was used as an internal control to evaluate the protoplast transfection efficiency. All the primers used for transient expression assay are listed in Supplementary Table 1 . Arabidopsis mesophyll protoplasts were prepared, transfected and cultured for 24 h before protein extraction and detection. Activities of GUS and luciferase were measured using microfluorometer (Cary Eclipse, USA). Relative GUS activity was calculated by normalizing against the luciferase activity, and the data presented were the averages of three biological replicates. Protein–DNA affinity pull-down assay The coding regions of yeast NF-YA (158-214aa) and yeast NF-YB (35-127aa) core domains for NF-Y combination [67] were cloned into the pQE30 vector to produce fusion proteins of His-Yeast NF-YA core and His-Yeast NF-YB, respectively. Primers used for constructions are listed in Supplementary Table 1 . His-NF-YC9 and GST-RGL2 fusion proteins were induced and purified as described above. Protein–DNA affinity assay was conducted with a modified method [68] . 1 μg of His-NF-YC9, 1 μg of His-Yeast NF-YA and 1 μg of His-Yeast NF-YB proteins were pre-incubated with various DNA fragments (0.5 μg each) produced by PCR using specific primes ( Supplementary Table 1 ) in the binding buffer (100 mM phosphate, 150 mM NaCl and 1 mM EDTA, pH 7.5) at 4 °C for 4 h. Then, the incubated protein–DNA samples were mixed with GST or GST-RGL2 immobilized by Glutathione Sepharose Beads (17-0756-01, Amersham Biosciences) at 4 °C for additional 4 h. After being washed with binding buffer three times, proteins and DNA retained on the beads were subsequently eluted by elution buffer (2% SDS, 50 mM Tris-HCl, 150 mM NaCl and 1 mM EDTA, pH 8.0) at 65 °C for 15 min twice, and the DNA pulled down was extracted and quantified by qPCR using specific primers ( Supplementary Table 1 ). The protein–DNA binding efficiency was calculated by normalizing the amount of DNA precipitated by proteins against that of the respective input DNA, and PP2A genomic DNA fragment was amplified and used as an internal control in this assay. The precipitated proteins bound to beads were detected by anti-His or anti-GST antibody as described above. Uncropped scans of western blot results are shown in Supplementary Fig. 16 . Data availability The RNA-seq data used in this study have been deposited in the Gene Expression Omnibus database under accession number GSE84753. All other data supporting the findings of this study are available within the article and its Supplementary Information files or on request from the corresponding author. How to cite this article: Liu, X. et al . The NF-YC–RGL2 module integrates GA and ABA signalling to regulate seed germination in Arabidopsis . Nat. Commun. 7:12768 doi: 10.1038/ncomms12768 (2016).